Imaging the post-fusion release and capture of a vesicle membrane protein The molecular mechanism responsible for capturing, sorting and retrieving vesicle membrane proteins following triggered exocytosis is not understood. Here we image the post-fusion release and then capture of a vesicle membrane protein, the vesicular acetylcholine transporter, from single vesicles in living neuroendocrine cells. We combine these measurements with super-resolution interferometric photo-activation localization microscopy and electron microscopy, and modelling to map the nanometer-scale topography and architecture of the structures responsible for the transporter’s capture following exocytosis. We show that after exocytosis, the transporter rapidly diffuses into the plasma membrane, but most travels only a short distance before it is locally captured over a dense network of membrane-resident clathrin-coated structures. We propose that the extreme density of these structures acts as a short-range diffusion trap. They quickly sequester diffusing vesicle material and limit its spread across the membrane. This system could provide a means for clathrin-mediated endocytosis to quickly recycle vesicle proteins in highly excitable cells. Cells of the nervous system communicate with one another by releasing peptides, neurotransmitters and other small molecules by exocytosis [1] . Once a vesicle has fused with the plasma membrane, the contents of the vesicle membrane can mix with the surface. These vesicular components must be recycled by endocytosis to maintain the size and molecular composition of the plasma membrane [2] . This process is called compensatory endocytosis. Two competing models for how cells accomplish this task have been proposed. These include the full-fusion model in which vesicle membrane components (proteins and lipids) diffuse laterally into the plasma membrane and are then captured far from exocytic sites by clathrin-mediated endocytosis, and the kiss-and-run model in which vesicles maintain their molecular composition, do not lose protein and lipid into the plasma membrane and are recaptured as intact organelles [3] , [4] . In this work we study the release and capture of a vesicle protein, the vesicular acetylcholine transporter (VAChT), from single synaptic-like microvesicles in neuroendocrine PC12 cells. Our results show that after triggered exocytosis, the transporter diffuses into the plasma membrane but more than half travels only several hundred nanometres before it is corralled over a dense network of endocytic structures. We propose that this housekeeping system could be used by cells to organize and maintain the composition of the plasma membrane during strenuous rounds of exocytosis. Imaging single synaptic microvesicles Here we imaged single synaptic-like microvesicles in living cells with total internal reflection fluorescence (TIRF) microscopy [5] . Specifically, we used a microvesicle-targeted pH-sensitive fluorescence probe (VAChT-pH) based on the VAChT ( Fig. 1a ) [6] . Single vesicles containing this probe brighten when the fusion pore of the vesicle opens after exocytosis and the acidic lumen of the vesicle is neutralized by the extracellular buffer [6] . 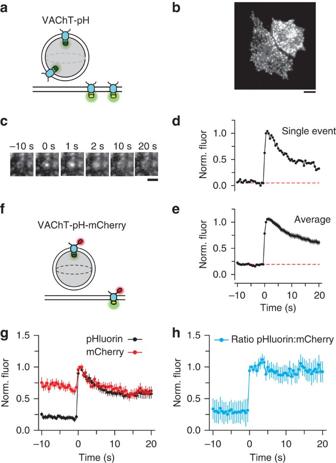Figure 1: Imaging single synaptic microvesicles in PC12 cells. (a) Cartoon of the microvesicle probe VAChT-pH. (b) Image of two PC12 cells expressing VAChT-pH imaged with TIRF. Scale bar equals 5 μm. (c) Frames from a movie where a single VAChT-pH-containing vesicle undergoes depolarization-triggered exocytosis, and (d) the corresponding fluorescence from the centre 750 nm-radius circle of that region. Scale bar equals 2 μm. (e) The mean VAChT-pH fluorescence from triggered exocytic vesicles (83 events, 13 cells). (f) Cartoon of the ratiometric pH probe VAChT-pH-mCherry. (g) The mean VAChT-pH-mCherry fluorescence from triggered exocytic vesicles in both the pHluorin and mCherry channels (36 events, 3 cells). The ratio of these two intensities is shown inh. Error bars are s.e.m. Norm. fluor., normalized fluorescence. Figure 1b shows two cells expressing VAChT-pH. Fluorescence was scattered across the bottom surface of the cell, where it was confined to small puncta. To test if these puncta were on the outside of the cell, we superfused cells with a low pH solution (pH 5.5; Supplementary Fig. S1 ). A dramatic dimming of the cells was measured during this treatment ( Supplementary Fig. S1a-c ). Single VAChT-pH puncta dimed and then re-brighted, indicating that many of the puncta were on the extracellular face of the plasma membrane. Some puncta did not dim, indicating that they were in intracellular compartments. To test if VAChT-pH was contained in acidic compartments, we superfused cells with ammonium chloride ( Supplementary Fig. S1d-f ). This chemical breaks down intracellular pH gradients. Cells and some fluorescent puncta exposed to this solution brightened, indicating that some VAChT-pH is located in intracellular acidic compartments ( Supplementary Fig. S1d-f ). Combined, these results indicate that VAChT-pH was present both in clusters on the plasma membrane and in acidic compartments within the cell. Figure 1: Imaging single synaptic microvesicles in PC12 cells. ( a ) Cartoon of the microvesicle probe VAChT-pH. ( b ) Image of two PC12 cells expressing VAChT-pH imaged with TIRF. Scale bar equals 5 μm. ( c ) Frames from a movie where a single VAChT-pH-containing vesicle undergoes depolarization-triggered exocytosis, and ( d ) the corresponding fluorescence from the centre 750 nm-radius circle of that region. Scale bar equals 2 μm. ( e ) The mean VAChT-pH fluorescence from triggered exocytic vesicles (83 events, 13 cells). ( f ) Cartoon of the ratiometric pH probe VAChT-pH-mCherry. ( g ) The mean VAChT-pH-mCherry fluorescence from triggered exocytic vesicles in both the pHluorin and mCherry channels (36 events, 3 cells). The ratio of these two intensities is shown in h . Error bars are s.e.m. Norm. fluor., normalized fluorescence. Full size image To evoke exocytosis, we depolarized cells with high potassium. This solution induced rapid and numerous exocytic events. Bright flashes could be seen across the bottom surface of the cell. These events were rare in unstimulated cells. Figure 1c shows an example event ( Supplementary Movie 1 ). Ten seconds before exocytosis, the vesicle is not visible, but when the fusion pore opens, a bright flash occurs within one frame (500 ms) and creates a bloom of fluorescence that radiates outward in all direction and dims ( Fig. 1c ). After exocytosis, some of this fluorescence was captured on preformed VAChT-pH clusters near the exocytic site ( Fig. 1c ). The fluorescence from the local membrane area (750 radius circle) surrounding this vesicle is plotted in Fig. 1d . This trace shows that VAChT-pH increases at exocytosis, decays within a few seconds and then plateaus to an intensity close to half of the peak value. The corresponding fluorescence from many events (83 events, 13 cells) is plotted in Fig. 1e . On average, VAChT-pH brightens rapidly and then decays. There is, however, a substantial amount of fluorescence (61±0.03%) that remains near the site of fusion ( Fig. 1e ). To determine if the VAChT-pH decay was due to loss of the protein into the plasma membrane (full-fusion) or was due to the direct recapture and re-acidification of the vesicle (kiss-and-run), we tagged VAChT-pH with mCherry. VAChT-pH-mCherry, positions the pH-sensitive pHluorin inside the vesicle lumen and the pH-insensitive mCherry into the cytoplasm ( Fig. 1f ). This sensor acts as a ratio-metric probe for pH changes in vesicles. The green fluorescence from VAChT-pH-mCherry rapidly brightens and then decays to 58±0.07% ( Fig. 1g ). Similarly, the mCherry fluorescence increases and then decays at the same rate, and to the same extent as pHluorin (62±0.07%; Fig. 1g ). The ratio of the red-to-green is shown in Fig. 1h , and shows that after exocytosis there is no change. Thus, the decay in VAChT-pH after exocytosis is not due to direct recapture and acidification (kiss-and-run), but instead is due to the loss of the probe into the membrane. These results support a full-fusion mechanism of exocytosis for VAChT. To analyse the spread of VAChT-pH, we measured four radial line scans centred over vesicles ( Fig. 2a ). These scans generated an average one-dimensional kymograph of the two-dimensional membrane surrounding exocytic events. 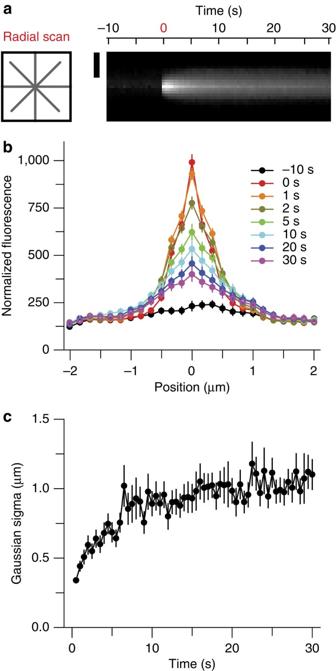Figure 2: Limited spread of VAChT-pH into the plasma membrane. (a) Mean normalized radial linescans of microvesicles during exocytosis (46 events, 13 cells). Scale bar equals 1.5 μm. (b) Intensity plot of the same radial linescans. (c) Meanσ-value of a Gaussian function fit to each of the events used foraandb. Error bars are s.e.m. Figure 2a shows results of averaging the kymographs of many VAChT-pH fusion events together. Upon exocytosis, fluorescence brightens and spreads rapidly. Fluorescence, however, progressed only a short distance. As seen in the example in Fig. 1c , some of the diffusing fluorescence remains near the site of fusion ( Fig. 2a ). The fluorescence from these kymographs is plotted in Fig. 2b . Analysis of these data is shown in Fig. 2c , where two-dimensional Gaussian functions were fit to vesicles. This plot shows that VAChT initially spreads rapidly, but remains relatively constant in size 10 s following exocytosis. We conclude that microvesicles release VAChT into the plasma membrane. Most of this material, however, does not spread more than a few hundred nanometres ( σ -values at 30 s, 1.1±0.1 μm) from the site of exocytosis. These results are consistent with several models of release for VAChT, which we consider below. Figure 2: Limited spread of VAChT-pH into the plasma membrane. ( a ) Mean normalized radial linescans of microvesicles during exocytosis (46 events, 13 cells). Scale bar equals 1.5 μm. ( b ) Intensity plot of the same radial linescans. ( c ) Mean σ -value of a Gaussian function fit to each of the events used for a and b . Error bars are s.e.m. Full size image Vesicle material is trapped in clathrin-coated structures The cytosolic tail of VAChT binds to the adaptor protein AP2 (refs 7 , 8 ). To determine if endocytic proteins were responsible for clustering vesicle material on the cell surface, and are involved in the retention of VAChT near sites of exocytosis, we imaged VAChT-pH together with two endocytic markers. 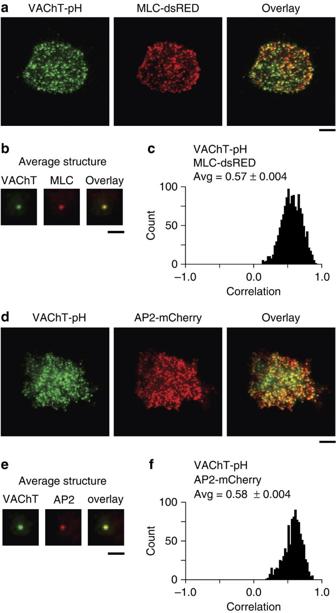Figure 3: VAChT-pH is clustered on endocytic proteins at the cell surface. (a) TIRF image of a cell co-expressing VAChT-pH and MLC-dsRED along with the overlay image. Scale bar equals 5 μm. (b) Mean extracted and normalized square regions centred on VAChT-pH spots and the corresponding regions from the MLC-dsRED channel (n=11 cells, 1,374 regions). Scale bar equals 2 μm. (c) The two-dimensional correlation values between the images used inb. (d) TIRF image of a cell co-expressing VAChT-pH and AP2-mCherry along with the overlay image. Scale bar equals 5 μm. (e) Mean extracted and normalized square regions centred on VAChT-pH spots and the corresponding region from the AP2-mCherry channel (n=6 cells, 964 regions). Scale bar equals 2 μm. (f) The two-dimensional correlation values between the images used ine. Avg, average. Figure 3a shows an image of VAChT-pH and a marker for clathrin-coated structures (clathrin light chain tagged with dsRED, mLC-dsRED) [9] . These images show that the bottom surface of PC12 cells have a large number of clathrin-coated structures (0.95 clathrin spots per μm 2 ±0.02 spots per μm 2 , n =11 cells, 79 regions (72 μm 2 area)). A similar density for clathrin was found with antibody staining ( Supplementary Fig. S2 ). To test if MLC-dsRED labelled all the clathrin structures, we immunostained cells expressing MLC-dsRED with antibodies against the heavy chain of clathrin. Almost all the antibody-stained clathrin spots were labelled with MLC-dsRED ( Supplementary Fig. S3 ). Furthermore, the number of antibody-stained clathrin structures was not increased compared with untransfected controls (X22 density of MLC-dsRED-transfected cells: 1.05±0.02 clathrin spots per μm 2 , X22 density of control cells: 1.06 clathrin spots per μm 2 ±0.03; Supplementary Figs S2 and S3 ). These results show that the density of clathrin was not changed by the expression of clathrin light chain ( Supplementary Figs S2 and S3 ). Figure 3: VAChT-pH is clustered on endocytic proteins at the cell surface. ( a ) TIRF image of a cell co-expressing VAChT-pH and MLC-dsRED along with the overlay image. Scale bar equals 5 μm. ( b ) Mean extracted and normalized square regions centred on VAChT-pH spots and the corresponding regions from the MLC-dsRED channel ( n =11 cells, 1,374 regions). Scale bar equals 2 μm. ( c ) The two-dimensional correlation values between the images used in b . ( d ) TIRF image of a cell co-expressing VAChT-pH and AP2-mCherry along with the overlay image. Scale bar equals 5 μm. ( e ) Mean extracted and normalized square regions centred on VAChT-pH spots and the corresponding region from the AP2-mCherry channel ( n =6 cells, 964 regions). Scale bar equals 2 μm. ( f ) The two-dimensional correlation values between the images used in e . Avg, average. Full size image When green images ( Fig. 3a ) were compared with red, a large fraction of VAChT-pH and clathrin colocalized ( Fig. 3a ). To analyse colocalization, we extracted 1,374 small (8.5 × 8.5 μm) images from 11 cells. In these regions, the centre of VAChT-pH structures were aligned to the middle pixel of the image. The corresponding regions from the MLC-dsRED image were also extracted. The fluorescence from these regions were normalized and averaged. This analysis showed a small distinct spot in the VAChT-pH image that co-localized with clathrin ( Fig. 3b ). The correlation between these regions is plotted in Fig. 3c and shows a strong and positive correlation. Visual inspection of 215 randomly chosen regions indicated that 85% of the central VAChT-pH spots had a corresponding signal in the MLC-dsRED channel. Similar analysis was done with VAChT-pH and AP2-mCherry ( Fig. 3d-f ). These images and their analysis show that, similar to clathrin VAChT-pH and AP2-mCherry strongly colocalize. Average VAChT-pH and AP2-mCherry image pairs have similar correlation values, sizes and distributions ( Fig. 3d-f ). Again, visual inspection of 215 randomly chosen regions showed that 82% of all the central VAChT-pH spots colocalized with AP2-mCherry. To test for the association of clathrin and AP2, we measured the colocalization of MLC-dsRED and AP2-green fluorescent protein (GFP; Supplementary Fig. S4 ). Visual inspection indicated that 98% of the MLC-dsRED had a corresponding signal in the AP2-GFP channel. Thus, almost all of the MLC-dsRED structures contained AP2-GFP. We conclude that there is a resting pool of VAChT-pH on the surface of the cell that is clustered on endocytic structures composed of clathrin and AP2. After exocytosis, vesicle material is trapped over clathrin We next asked if the corralling of VAChT-pH observed after exocytosis is related to clathrin. To answer this question, we triggered exocytosis in cells expressing VAChT-pH and MLC-dsRED. We then imaged the release of VAChT-pH from single exocytic vesicles and compared these images with clathrin. 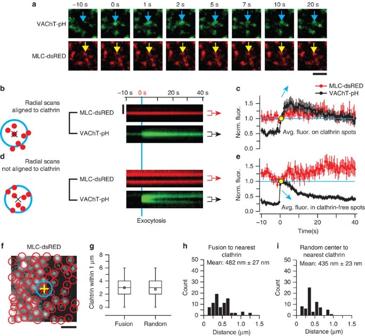Figure 4: VAChT-pH is captured by preformed clathrin structures after exocytosis. (a) Sequential two-colour TIRF images of a single vesicle fusing with the plasma membrane. The location of fusion is indicated by the blue arrow. After fusion, VAChT-pH is captured on a preformed clathrin-coated pit (yellow arrow) located close to the site of exocytosis. Scale bar equals 2 μm. (b) Mean radial linescans through images centred on clathrin structures located within 1 μm of an exocytic event (n=7 cells, 35 regions). Fusion occurs at zero seconds. Scale bar equals 2 μm. (c) The measured fluorescence from VAChT-pH and MLC-dsRED from a circle with a radius of 375 nm centred on the clathrin structures shown inb. (d) Mean radial linescans through images centred on clathrin-free areas located within 1 μm of an exocytic event (n=7 cells, 43 regions). (e) The measured fluorescence from VAChT-pH and MLC-dsRED from a circle with a radius of 375 nm centred on the centre of the clathrin-free areas shown ind. Spatial analysis comparing sites of exocytosis (f, yellow cross) to clathrin (f, red circles). Scale bar equals 2 μm. The blue circle indicates an area 1 μm from the centre of exocytosis. (g) Plot of the number of clathrin structures located within 1 μm of fusion events (n=11 cells, 79 regions, 4,383 clathrin structures). (h) Histogram showing nearest-neighbour distances between fusion sites and clathrin spots. (i) Histogram showing the nearest-neighbour distances between random sites and clathrin spots. Error bars are s.e.m. Avg. fluor., average fluorescence; Norm. fluor., normalized fluorescence. Figure 4a shows a single exocytic vesicle arriving at the surface and rapidly brightening. VAChT-pH left the site of exocytosis and diffused radially into the plasma membrane where a fraction of the fluorescence was rapidly (<1 s) captured on a preformed clathrin structure ( Fig. 4a ; Supplementary Fig. S5 and Supplementary Movie 2 ). This trapped VAChT-pH remained associated with clathrin for over 20 s. Figure 4: VAChT-pH is captured by preformed clathrin structures after exocytosis. ( a ) Sequential two-colour TIRF images of a single vesicle fusing with the plasma membrane. The location of fusion is indicated by the blue arrow. After fusion, VAChT-pH is captured on a preformed clathrin-coated pit (yellow arrow) located close to the site of exocytosis. Scale bar equals 2 μm. ( b ) Mean radial linescans through images centred on clathrin structures located within 1 μm of an exocytic event ( n =7 cells, 35 regions). Fusion occurs at zero seconds. Scale bar equals 2 μm. ( c ) The measured fluorescence from VAChT-pH and MLC-dsRED from a circle with a radius of 375 nm centred on the clathrin structures shown in b . ( d ) Mean radial linescans through images centred on clathrin-free areas located within 1 μm of an exocytic event ( n =7 cells, 43 regions). ( e ) The measured fluorescence from VAChT-pH and MLC-dsRED from a circle with a radius of 375 nm centred on the centre of the clathrin-free areas shown in d . Spatial analysis comparing sites of exocytosis ( f , yellow cross) to clathrin ( f , red circles). Scale bar equals 2 μm. The blue circle indicates an area 1 μm from the centre of exocytosis. ( g ) Plot of the number of clathrin structures located within 1 μm of fusion events ( n =11 cells, 79 regions, 4,383 clathrin structures). ( h ) Histogram showing nearest-neighbour distances between fusion sites and clathrin spots. ( i ) Histogram showing the nearest-neighbour distances between random sites and clathrin spots. Error bars are s.e.m. Avg. fluor., average fluorescence; Norm. fluor., normalized fluorescence. Full size image To analyse the capture of VAChT-pH on clathrin, we measured fluorescence around clathrin structures located within1 μm of fusion events. The average kymographs centred over clathrin is shown in Fig. 4b . From this analysis, it is evident that clathrin is stable at the membrane before exocytosis. At the moment of fusion, VAChT-pH brightens in the membrane area surrounding clathrin, steadily increases and is then focused onto the central clathrin-containing spot ( Fig. 4b ). We observe that the width of the VAChT-pH spot decrease after exocytosis and aligns with the central spot of clathrin in the kymograph ( Fig. 4b ). A plot of the fluorescence intensity during exocytosis measured in a small membrane area (375 nm radius circle) over clathrin is shown in Fig. 4c . In these clathrin-containing regions, VAChT-pH fluorescence steadily increases after exocytosis and then plateaus ( Fig. 4c ). The small and slow decline of fluorescence over clathrin during the plateau phase could be due to several experimental issues, including photobleaching, vesicle movement, re-acidification and endocytosis. These data demonstrate that the trapping of VAChT-pH occurs over resident clathrin structures located within a micron of exocytosis. To show that VAChT-pH is specifically trapped over clathrin after exocytosis, we measured VAChT-pH in regions that did not contain clathrin and were located within 1 μm of fusion events. The average kymograph centred over clathrin-free areas is shown in Fig. 4d . In these regions, VAChT-pH brightens at exocytosis and is then rapidly lost. Specifically, VAChT-pH diffuses from the central, clathrin-free area, and is then captured on the surrounding clathrin. Unlike Fig. 4c , the fluorescence from clathrin-free areas (375 nm radius circle) increases at exocytosis, does not continue to increase and then rapidly decays ( Fig. 4e ). These data demonstrate that after exocytosis, VAChT-pH freely diffuses in membranes that do not contain clathrin, and is caught on membranes that do contain clathrin. To test for a spatial coupling between sites of exocytosis and endocytosis, we mapped the location of 79 exocytic vesicles in relation to all clathrin spots. Figure 4f shows an example image of a field of clathrin where an exocytic event occurs in the centre ( Fig. 4f , yellow cross). For this analysis, we determined the location of all the clathrin structures in each image surrounding exocytic sites (11 cells, 79 regions, 4,383 spots). The same analysis was done for control images from the same cells (7 cells, 67 images, 3,941 spots). This analysis shows that there is a dense network of clathrin across the cell surface. Interestingly, there was no increase in the number of clathrin structures near sites of exocytosis (2.9 spots±0.2 spots) compared with the control images (2.7 spots±0.2 spots; Fig. 4g ). A histogram showing the distance between exocytic sites and the closest clathrin structure is plotted in Fig. 4h . The closest clathrin structure to each fusion site was 482±27 nm. Figure 4i shows that the nearest-neighbour spacing of clathrin structures is 706±11 nm (4,373 structures, 79 regions, 11 cells). For controls, the clathrin structure nearest to the centre of the image was 435±23 nm and the nearest-neighbour spacing of clathrin was 711±11 nm. Thus, material exiting a vesicle needs to go no further than a few hundred nanometres before it encounters a preformed clathrin structure. This distribution of clathrin, however, is not linked to sites of exocytosis. Instead, it is randomly generated by the spacing and high density of resident clathrin structures. To support the hypothesis that classical clathrin-mediated endocytosis was linked to the surface distribution of VAChT, we treated cells with the dynamin inhibitor dynasore [10] . Like MLC-dsRED and AP2-mCherry, Dynamin1-mCherry (Dyn1-mCherry) co-localized with VAChT-pH ( Supplementary Fig. S6 ). Visual inspection indicated that 64% of VAChT-pH spots co-localized with Dyn1-mCherry spots ( Supplementary Fig. S6 ). When cells were exposed to 80 μM dynasore for 30 min, a dramatic increase in surface fluorescence over time was observed ( Supplementary Fig. S6 ). This increase in fluorescence occurred in both the stable fluorescent puncta and plasma membrane regions not associated with puncta. Thus, the surface distribution and recycling of VAChT-pH is dependent on the action of components of clathrin-coated pits, namely dynamin. Architecture of clathrin determined by iPALM From the above data, we conclude that a large fraction of vesicle material is rapidly and locally captured over pre-formed clathrin structures after triggered exocytosis. Standard optical microscopy (for example, TIRF) is restricted by the diffraction limit of light. This fact limits the resolution of cellular structures to ~200 nm with TIRF. Thus, we used a super-resolution optical technique known as interferometric photo-activation localization microscopy (iPALM) to image the three-dimensional sub-diffraction size and distribution of clathrin in PC12 cells [11] . To accomplish this, we tagged clathrin light chains with the photo-switchable fluorescent protein mEOS2 (mLC-mEOS2; Fig. 5a ) [12] . iPALM was used to reconstruct the size, shape and distribution of clathrin at the bottom surface of the plasma membrane. iPALM also allows one to analyse the distribution of clathrin molecules in the plane perpendicular to the coverslip [11] . 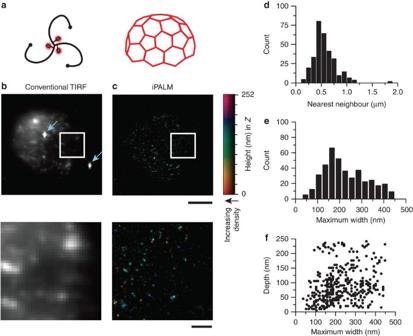Figure 5: iPALM measurements of clathrin shape and density. (a) Cartoon of a single clathrin triskeleon with a light chain labelled with a fluorescent protein. The triskeleons assemble together to form clathrin-coated structures. (b) Conventional TIRF optical image and (c) iPALM measurement of MLC-mEOS2 in a PC12 cell. Scale bar equals 5 μm. Inb, the blue arrows point to gold particles used for alignment. In both cases, a magnified view of the white box is shown below. Scale bar equals 1 μm. (d) Histogram of clathrin spacing in PC12 cells measured with iPALM. (e) Histogram showing the width of the same structures. (f) Plot of width versus depth of the clathrin objects measured with iPALM. Error bars are s.e.m. Figure 5b shows a single cell imaged with iPALM. The images to the left shows the cell imaged with a conventional TIRF, and to the right shows the same cell imaged with iPALM. Clearly, individual spots of clathrin are difficult to distinguish with conventional imaging. However, distinct clathrin structures are clearly visible with iPALM. Figure 5: iPALM measurements of clathrin shape and density. ( a ) Cartoon of a single clathrin triskeleon with a light chain labelled with a fluorescent protein. The triskeleons assemble together to form clathrin-coated structures. ( b ) Conventional TIRF optical image and ( c ) iPALM measurement of MLC-mEOS2 in a PC12 cell. Scale bar equals 5 μm. In b , the blue arrows point to gold particles used for alignment. In both cases, a magnified view of the white box is shown below. Scale bar equals 1 μm. ( d ) Histogram of clathrin spacing in PC12 cells measured with iPALM. ( e ) Histogram showing the width of the same structures. ( f ) Plot of width versus depth of the clathrin objects measured with iPALM. Error bars are s.e.m. Full size image From images of entire cells, we were able to calculate the sub-diffraction distribution of clathrin. The total density of resolvable spots was 2.00±0.09 spots per μm 2 (3 cells). Nearest-neighbour analysis showed that the average spacing was 560±1 nm ( n =3 cells, 305 spots; Fig. 5d ). This was 200 nm closer than we observed with conventional TIRF. To systematically analyse the shape of all the structures on the surface, we measured the width and depth of each structure from three cells in the x, y and z dimensions relative to the glass coverslip. Figure 5e shows that the size of clathrin-coated structures ranged from 50 to 450 nm in diameter (mean: 224±5 nm, n =3 cells, 401 structures). These structures varied in shape with 42% less than 75 nm in depth ( Fig. 5f ). From these measurements, there was no strong correlation between the width and depth of individual pits. These data support the finding that the density of clathrin structures in these cells is very high. Furthermore, individual structures were either flat or domed. The functional importance of these two types of structures is yet to be determined. Finally, the two-fold increase in density observed with iPALM can be explained by the inability of traditional optical imaging (TIRF) to delineate between two closely spaced structures and one large structure. Architecture of clathrin determined by electron microscopy To further map the architecture of clathrin, we performed electron microscopy. We first prepared platinum-shadowed membrane sheets from PC12 cells [13] . We then used whole-cell transmission electron microscopy to visualize the entire inner surface of the plasma membrane ( Supplementary Fig. S7 ). We observed two types of clathrin structures: (1) distinctive flat patches and (2) domes, or pit-like structures ( Supplementary Movie 3 ). 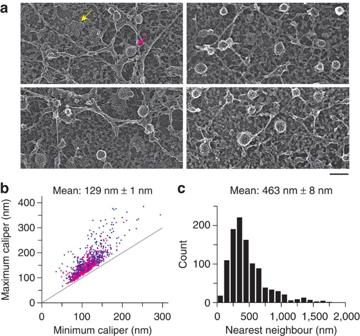Figure 6: Shape and density of clathrin structures measured with electron microscopy. (a) Four representative transmission electron microscopic images of the inner surface of the plasma membrane of PC12 cells. A representative flat (yellow arrow) and domed (pink arrow) structure are indicated. Scale bar equals 200 nm. (b) Plot of minimum and maximum caliper measurement for all visible clathrin structures over the entire cell (n=3 cells, 64 regions, 1,045 clathrin structures). Pink circles are structures classified as domed and purple circles are structures classified as flat. (c) Nearest-neighbour analysis of all the clathrin structures shown inb. Figure 6a shows four regions where both flat patches and pits of clathrin can be seen. To determine the shape of these structures, we measured the minimum and maximum dimension (1,045 clathrin structures, 96 regions, 3 cells). The structures were further classified by eye as flat or domed. Figure 6b shows a scatter plot of these measurements. The structures have a maximum diameter of 129±1 nm (1,045 clathrin structures, 96 regions, 3 cells). Figure 6c show this nearest-neighbour analysis. Clathrin structures were distributed at a nearest-neighbour density of 463±8 nm (3 cells). The total density was 1.6 clathrin structures per μm 2 ±0.11 (96 regions, 3 cells). To further confirm these densities, we performed super-resolution imaging ( Supplementary Fig. S8 ). The density observed with ground-state depletion (GSD) imaging showed 2.3 structures per μm 2 ±0.08 (92 regions, 6 cells). Again, these data support the finding that the density of clathrin on the surface is very high, between 2 and 11 times greater than previously reported from other cell types [14] , [15] , [16] , [17] , [18] , [19] , [20] . Furthermore, these data demonstrate that the density of clathrin structures measured in iPALM was not a consequence of overexpression. The differences between our EM, iPALM and GSD-measured clathrin densities likely resulted from the systematic measurement errors of each method. For example, some clathrin structures are hidden by other cellular structures in our EM images. Furthermore, background fluorescence could result in a slight overcounting of clathrin structures in iPALM and GSD imaging. These measurements support the model in which fusion occurs randomly among sites of endocytosis, and diffusing material can be rapidly captured on preformed clathrin-coated structures waiting on the cell surface to trap material destined for endocytosis. Figure 6: Shape and density of clathrin structures measured with electron microscopy. ( a ) Four representative transmission electron microscopic images of the inner surface of the plasma membrane of PC12 cells. A representative flat (yellow arrow) and domed (pink arrow) structure are indicated. Scale bar equals 200 nm. ( b ) Plot of minimum and maximum caliper measurement for all visible clathrin structures over the entire cell ( n= 3 cells, 64 regions, 1,045 clathrin structures). Pink circles are structures classified as domed and purple circles are structures classified as flat. ( c ) Nearest-neighbour analysis of all the clathrin structures shown in b . Full size image Modelling To test the hypothesis that a dense field of traps can limit the spread of VAChT, we developed a simple physical model ( Fig. 7a ). First, particles in the centre of a small field were allowed to undergo random two-dimensional Brownian diffusion. These simulations were observed to lose all the particles rapidly ( Fig. 7b and Supplementary Movie 4 ). When we introduced a population of traps into the simulation (1, 2 and 5 traps per μm 2 ), we observe a rapid capture of particles near sites of release ( Fig. 7b and Supplementary Movie 5 ). The amount of capture was directly related to the density of traps. This is observed in Fig. 7b and Supplementary Movie 5 . A plot measuring the fluorescence from simulations shows that without traps fluorescence is rapidly lost from the centre (750 nm radius region) into the surrounding membrane ( Fig. 7c ). The plot, however, of average simulations that included traps shows a rapid loss and then a plateau of fluorescence ( Fig. 7c ). The size of the plateau is proportional to the number of traps. These simulations support the hypothesis that a dense network of traps can account for the limited spread and rapid capture of VAChT. Furthermore, the density of traps can modulate the amount of material lost or remaining near any individual site of release. 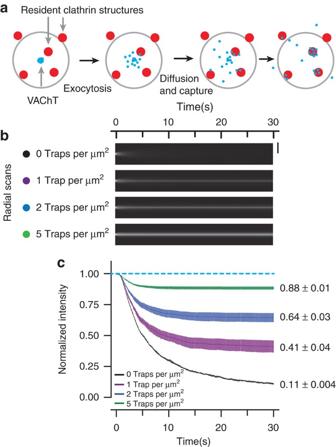Figure 7: A simple model for exocytic recapture. (a) Cartoon of the model for the release and capture of VAChT. (b) Radial kymograph of fluorescence from the mean of five diffusion simulations. The simulations contained 0, 1, 2 and 5 traps per μm2. The material rapidly exits the centre, but a large amount of the particles are caught and remain in the centre in simulations that contain traps. Scale bar equals 2 μm. (c) Plot of the mean intensity contained in circular regions with a radius of 750 nm from the above simulations. Error bars are s.e.m. Figure 7: A simple model for exocytic recapture. ( a ) Cartoon of the model for the release and capture of VAChT. ( b ) Radial kymograph of fluorescence from the mean of five diffusion simulations. The simulations contained 0, 1, 2 and 5 traps per μm 2 . The material rapidly exits the centre, but a large amount of the particles are caught and remain in the centre in simulations that contain traps. Scale bar equals 2 μm. ( c ) Plot of the mean intensity contained in circular regions with a radius of 750 nm from the above simulations. Error bars are s.e.m. Full size image Here we image the dynamic architecture of release and capture of a vesicle membrane protein. When vesicles fuse with the plasma membrane, VAChT diffused into the plasma membrane within a second. This supports a full-fusion model of exocytosis. A portion of this material, however, was then trapped over a dense matrix of endocytic structures. We propose that the density of these resident clathrin-containing structures ensured that most of the transporter did not diffuse more than several hundred nanometres in the plasma membrane. We further mapped the distribution and architecture of these structures with super-resolution and electron microscopy. These measurements showed a dense network of clathrin structures that coated the inner plasma membrane. Finally, modelling supports the idea that a simple system of randomly distributed traps at high density can account for the limited spread of vesicle material and its rapid capture. In excitable cells, experiments have supported two modes of vesicle recapture. First, work in neurons has suggested that during exocytosis vesicles collapse into the plasma membrane and material is retrieved at sites distant from exocytic sites [21] , [22] , [23] . Retrieval has been suggested to occur by the assembly of clathrin onto vesicle material [24] . Other work has suggested that vesicles might instead rapidly open and close a narrow fusion pore, losing no lipids and no protein [25] , [26] , [27] . Past work has suggested that this mechanism (kiss-and-run) might be the dominant mode of fusion for synaptic-like microvesicles [28] . Modified forms of these models have been proposed. For example, studies have suggested that some proteins released from vesicles can remain as patches on the cell surface [29] , [30] . These clusters could provide platforms for the efficient recapture of vesicle material and the rapid rebuilding of new vesicles [31] , [32] , [33] . In PC12 cells and chromaffin cells, large dense-core granules have been observed to fuse with the membrane, but not release membrane proteins [34] , [35] . These partially empty granule cavities were then observed to be directly recaptured [34] , [35] , [36] , [37] . Here, in PC12 cells we observe a different mechanism for the release of VAChT from small synaptic-like microvesicles. Transporters that exit the vesicle during a full-fusion-type exocytosis are rapidly captured on endocytic traps close to sites of exocytosis. Thus, different mechanisms of vesicle recycling can operate in different vesicle populations within the same cell. The organization of endocytic zones in PC12 cells is similar to structures seen in neurons. For example, in neuromuscular junctions, endocytic zones have been seen to surround sites of exocytosis [38] , [39] . This organization has been proposed to provide a mechanism to rapidly capture vesicle proteins. Classical clathrin-mediated endocytosis has been proposed to be too slow to keep pace with the sometimes high rates of exocytosis in excitable cells [3] . If exocytosis outruns endocytosis, the accumulation of vesicle material on the cell surface would be harmful to the continued function of the cell. Here we show that vesicle transporters lost into the membrane can be rapidly captured over a dense matrix of resident clathrin structures. Other than clathrin and AP2, alternative proteins within these domains including clathrin-associated cytoskeletal elements, or membrane proteins, could also be responsible for slowing the diffusion of VAChT. Future work is needed to determine the specific molecules responsible for capturing VAChT over clathrin microdomains. Plasmids, solutions and cells VAChT-pH was a gift from D. Clapham (Harvard) [6] . VAChT-pH-mCherry was made by cloning mCherry behind the carboxy-terminal tail of VAChT-pH. MLC-mEOS2 was made by replacing dsRED with mEOS2 in MLC-dsRED [9] . mEOS2 was a gift from C. Waterman (NHLBI). AP2-mCherry (rat μ-subunit) and Dyn1-mCherry were gifts from C.J. Merrifield (CNRS). AP2-GFP was a gift of Lois Greene (NHLBI). Dyn-GFP was described previously [9] . ITPKA-tdTomato was a gift from M. Schell (Uniform Services University). PC12-GR5 cells were cultured as described [34] , [35] . Cells were plated onto poly ( L -lysine)-coated glass coverslips. Cells were transfected with 1 μg of plasmid using Lipofectamine 2,000 (Invitrogen). For imaging, cells were maintained in buffer (130mM NaCl, 2.8mM KCl, 5mM CaCl 2 , 1mM MgCl 2 , 10mM HEPES, 10mM glucose, pH 7.4). To stimulate exocytosis, cells were depolarized with elevated [K + ] (105mM KCl, 50mM NaCl, 2mM CaCl 2 , 0.7mM MgCl 2 , 1mM NaH 2 PO 4 , 10mM HEPES, pH 7.4). In some experiments, cells were perfused with a low pH solution (130mM NaCl, 2.8mM KCl, 5mM CaCl 2 , 1mM MgCl 2 , 10mM MES, 10mM glucose, pH 5.5) or ammonium chloride (80mM NaCl, 50mM NH4Cl, 2.8mM KCl, 5mM CaCl 2 , 1mM MgCl 2 , 10mM HEPES, 10mM glucose, pH 7.4) through a microperfusion system (μ-flow 8, ALA Scientific). Experiments were carried out at 30 °C. TIRF microscopy Cells were imaged with an inverted microscope (IX-81; Olympus) configured for TIRF with a X100, 1.45 numerical aperture (NA) objective (Olympus) and an image splitter (Photometrics). Fluorescence was excited by 488 nm laser (Melles Griot series 43 ion laser) and 561 nm laser (Melles Griot LD-561-20A). Lasers were combined and controlled with an acousto-optic tunable filter (Andor). Filters were bright-line full multiband LF405/488/561/635 filters (Semrock). The resulting emission was then divided by the image splitter’s dichroic (565DCXR) and projected side-by-side through 525Q/50 and 605Q/55 emission filters onto the chip of an EMCCD camera (Andor DU 897). Images were acquired using the IQ software (Andor). For alignment of the red and green images, we imaged 100 nm fluorescent beads (Invitrogen) that emitted light in both the red and green channels. Regions were aligned by matching the bead locations between the two regions. Pixel size was 167 nm. Frames were acquired with alternating 488 and 561 nm excitation (100 ms exposures at 2 Hz). TIRF analysis Analysis was done in Metamorph (Molecular Devices) or MATLAB (Mathworks). For co-localization, green objects were centred in an 8.5 × 8.5-μm region with a custom automated programme written in MATLAB. Images were excised and normalized to the brightest pixel and averaged. The corresponding red images were excised and normalized to the brightest pixel and averaged. To locate exocytic events, movies were scanned for brightening events. Events were identified that showed a rapid brightening in a diffraction-limited spot that occurred within one frame. The time and location of each event was catalogued and small regions (8.5 × 8.5 μm) were excised as stacks. Only events that occured 2 μm or more from the edge of the cell were used. Onset of exocytosis was defined as the first frame showing a visible increase in fluorescence over background. In two-colour experiments, regions located in the green image were transferred to the corresponding red image. Fluorescence was measured in a 1.5 μm-diameter circle centred on the vesicle. These traces were normalized to the frame 0.5 s after the start of exocytosis. Analysis of clathrin and clathrin-free membrane areas used 750-nm diameter circles. To generate radial kymographs, a custom written MATLAB programme was used to measure linescans of 4.1 μm in length arrayed as a star pattern. These scans were averaged to generate an average kymograph through time. To fit two-dimensional Gaussians, a custom written MATLAB programme was used. For analysis of clathrin density, MLC-dsRED expressing cells were scanned for clathrin spots. Individual spots were marked and their Cartesian co-ordinates catalogued. These locations were used to calculate distances. iPALM We used the iPALM method described in Shtengel et al. [11] with a z axis distance range of 750 nm [40] . First, 25 × 35 nm bare Au nanorods (part number 30-25-550, Nanopartz) were deposited onto 25 mm, number 1.5 coverslips (Warner Instruments). Next, a 50-nm layer of SiO 2 was sputtered over the top of the Au-coated coverslips using a Denton Explorer sputtering system (Denton Vacuum). For imaging, cells grown on these coverslips were fixed with 2% paraformaldehyde in PHEM butter (25 mM HEPES, 10 mM EGTA, 60 mM PIPES, 2 mM MgCl 2 , pH 7) for 15 min. Next, 18 mm, number 1.5 coverslip was mounted over the cells and sealed. Typical acquisition consisted of 40,000–60,000 frames under 561 nm illumination (power density ~2 kW cm −2 ). The exposure time was 50 ms. Photo-activation was done during the readout phase with 5–25 ms pulses of 405 nm illumination (power density 2–10 W cm −2 ). Au nanoparticles were used for calibration and drift correction. Calibration and data analysis have been described [11] , [40] . For processing, individual molecules were identified in custom software written in IDL (ITT Vis). Collections of molecules were analysed as individual structures by finding their centres of mass and dimensions in the X, Y and Z planes. Electron microscopy Cells were stabilized with a hypotonic poly-lysine solution in PBS for 30 s and sonicated in stabilization buffer (70 mM KCl, 30 mM HEPES, 5 mM MgCl2, 3 mM EGTA, 1 mM DTT, protease inhibitor cocktail) for 1 s with a Branson 450 sonicator using a 3-mm metal tip positioned 1 cm above the coverslip. Membranes were fixed in 2% glutaradehyde in stabilization buffer for 4 h at room temperature. Samples were rinsed with de-ionized water, fixed and stained with 0.1% aqueous uranyl acetate for 20 min at room temperature. Samples were rinsed with water and dehydrated in 5 min steps in a graded ethanol series (% in water): 15, 30, 50, 70, 80, 90, 100 twice, 100 stored over Molecular Sieve (EM Science) twice. The dehydrated samples were dried out of liquid CO 2 at the critical point in a Samdri-795 critical point dryer (Tousimis) and transferred to the stage of a JEOL RFD9010 freeze-fracture device (RMC-Boeckler) where they were rotary shadowed with platinum at an angle of 17° for 12 s, and coated with carbon at an angle of 80° for 12 s. The replicas were scored into pieces ~2 mm 2 , released by floatation on 10% HF, rinsed in water, cleaned with 50% Clorox, water rinsed and mounted on 150-mesh formvar-coated copper grids and imaged at X30,000 with a JEM 1400 electron microscope (JEOL USA Inc.) operating at 120 kV and equipped with an AMT XR-111 digital camera (Advanced Microscopy Techniques). Montages consisting of 36 tiled images were acquired at X15,000 using Serial EM (Boulder Laboratory for 3-D Electron Microscopy of Cells, University of Colorado). Modelling Simulations were performed in MATLAB. One hundred particles started at the origin. Each particle took random steps in both the x and y co-ordinates according to Brownian dynamics where X i =(x i,j , y i,j ) is the position of the j th particle after i steps, W i is a vector of random values with a standard normal distribution, D is the diffusion coefficient and Δ t is the time step. For simulations, D =0.04 μm 2 s −1 and Δ t =8 × 10 −5 s. This diffusion coefficient was chosen, because it lies between the two diffusion co-efficients measured for syntaxin in PC12 cells [41] , [42] . Each particle took 5 × 10 5 steps (40 s of simulation). To simulate clathrin traps, 100 nm diameter traps were randomly placed at a specified density (0, 1, 2 or 5 traps μm −2 ) in a 20 × 20-μm 2 region around the origin. If a particle took a step into the trap, it became stationary. Every 0.1 s, the positions were converted into an image by making a two-dimensional histogram with 0.01 × 0.01 μm bins. The images were then convolved with a two-dimensional Gaussian ( σ x,y =0.21 λ /NA) approximating the point spread function of the microscope, where λ =0.5 μm is the approximate wavelength of light and NA=1.45 is the numerical aperture of the microscope objective. Finally, images were binned to obtain pixel sizes of 0.1 × 0.1 μm. How to cite this article: Sochacki, K. A. et al. Imaging the post-fusion release and capture of a vesicle membrane protein. Nat. Commun. 3:1154 doi: 10.1038/ncomms2158 (2012).